MPIase is a glycolipozyme essential for membrane protein integration Protein integration into biological membranes is a vital cellular event for all organisms. We previously reported an integration factor in the inner membrane of Escherichia coli , named MPIase (membrane protein integrase). Here we show that in contrast to previously identified integration factors that are proteins, MPIase is a glycolipid composed of diacylglycerol and a glycan chain of three acetylated aminosugars linked through pyrophosphate. Hydrolytic removal of the lipid moiety gives a soluble product with higher integration activity than that of the original MPIase. This soluble form of MPIase directly interacts with a newborn membrane protein, maintaining its integration-competent structure and allowing its post-translational integration. MPIase actively drives protein integration following chaperoning membrane proteins. We further demonstrate with anti-MPIase antibodies that MPIase is likely involved in integration in vivo . Collectively, our results suggest that MPIase, essential for membrane protein integration, is to our knowledge the first glycolipid with an enzyme-like activity. Membrane proteins possessing water-insoluble membrane-spanning regions are integrated into biological membranes co-translationally. The fundamental mechanisms underlying protein integration are conserved in all organisms, in which signal recognition particles (SRP) and protein-conducting channels (SecYEG in bacteria and Sec61 in eukaryotes) are utilized to support co-translational integration [1] , [2] , [3] ( Supplementary Fig. S1 ). Besides, a Sec/SRP-independent pathway has been shown to be present in both Escherichia coli ( Supplementary Fig. S2 ) and eukaryotic cells, as a subset of small-membrane proteins and tail-anchored (TA) membrane proteins are unable to utilize the SRP system [4] , [5] , [6] . This pathway has been considered to be a spontaneous process operated by hydrophobic interactions between a membrane-spanning region and membrane lipids in E. coli , whereas chaperones required for membrane targeting of TA proteins have been identified in eukaryotes [6] , [7] , [8] . With this background, we recently proved that this process in E. coli is also regulated by membrane components. The first clue to this achievement was our previous observation that the physiological concentration of diacylglycerol (DAG), when present in liposomes, blocks spontaneous integration of Sec/SRP-independent substrates [9] , [10] ( Supplementary Fig. S3 ). Spontaneous integration then turned out to be an artificial event judging from the fact that even Sec/SRP-dependent substrates were integrated into liposomes without the aid of Sec proteins in the absence of DAG [9] . No spontaneous integration of Sec/SRP-dependent substrates occurs in DAG-containing liposomes mimicking biomembranes, even if they have been solubilized with SRP [9] . We subsequently found that the addition of an extract of cell membranes to DAG-containing liposomes restored the integration [9] . Therefore, the presence of an unknown factor, to be called ‘membrane protein integrase’, in cell membranes was strongly suggested. We attempted to isolate the factor from inner membranes of E. coli. A new factor giving an 8 kDa band on a urea/SDS gel was successfully purified [11] . The factor proved to be indispensable in both Sec/SRP-dependent and -independent manners [9] , [10] , [11] . We named it MPIase ( m embrane p rotein i ntegr ase ) after its function [11] ; however, its structure was totally unknown. Although a derivative of lipid A, the lipid part of lipopolysaccharides [12] had been suggested to be the factor in the process of purification [9] , and later extensive purification proved that this was not the case [11] . Here, we report the complete structural study and functional characterization of MPIase. Surprisingly, MPIase is a new glycolipid possessing integration-dedicated chaperone-like activity that drives subsequent membrane integration. Thus, the enzyme-like activity of MPIase leads us to propose that MPIase is the first example of a ‘glycolipozyme’. Determination of the MPIase structure We determined the MPIase structure ( Fig. 1a ) as follows. Highly purified MPIase [11] obtained from inner membrane vesicles (INV) of E. coli was used for the following experiments. On amino-acid analysis after HCl hydrolysis, MPIase gave only two peaks corresponding to glucosamine and ammonia, that is, none of the amino acids, suggesting that MPIase is non-proteinaceous and consists of unstable aminosugars. Capillary gas chromatography-mass spectrometry (GC–MS) analysis after methanolysis of MPIase demonstrated the presence of fatty acids, suggesting that MPIase is a glycolipid. 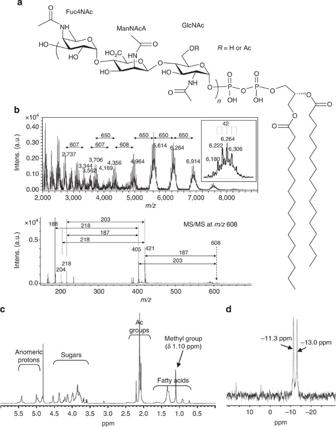Figure 1: Determination of the MPIase structure. (a) Structure of MPIase n=7–14 (mainly 9–11). (b, top) MALDI–TOF MS spectrum of MPIase in the negative mode. Subdivided peaks differing in 42 mass units reflect variation ofO-acetyl groups. (Bottom) The MS/MS spectrum fromm/z608 in the positive mode contained fragment peaks comprising combinations of 187, 203 or 217 mass units. (c) A1H-NMR spectrum of MPIase (750 MHz, D2O) indicates the presence of a methyl group,N-acetyl groups, anO-acetyl group, fatty acids and sugar moieties. (d)31P-NMR spectrum of MPIase measured on a Bruker DMX-500 spectrometer. The chemical shifts relative to 5% H3PO4of these two peaks indicate the presence of a diester of pyrophosphate15. a.u., arbitrary unit. Figure 1: Determination of the MPIase structure. ( a ) Structure of MPIase n=7–14 (mainly 9–11). ( b , top) MALDI–TOF MS spectrum of MPIase in the negative mode. Subdivided peaks differing in 42 mass units reflect variation of O -acetyl groups. (Bottom) The MS/MS spectrum from m/z 608 in the positive mode contained fragment peaks comprising combinations of 187, 203 or 217 mass units. ( c ) A 1 H-NMR spectrum of MPIase (750 MHz, D 2 O) indicates the presence of a methyl group, N -acetyl groups, an O -acetyl group, fatty acids and sugar moieties. ( d ) 31 P-NMR spectrum of MPIase measured on a Bruker DMX-500 spectrometer. The chemical shifts relative to 5% H 3 PO 4 of these two peaks indicate the presence of a diester of pyrophosphate [15] . a.u., arbitrary unit. Full size image Matrix-assisted laser desorption/ionization time-of-flight mass spectrometry (MALDI-TOF MS) of MPIase showed a series of peaks over m/z 4,000 ( Fig. 1b , top). A definite molecular formula could not be determined at this stage because of the presence of such multiple peaks and insufficient resolution of isotopic peaks. The presence of many peaks with 42 mass unit intervals indicates various extents of acetylation in the molecule. Moreover, the characteristic repeating pattern with 608 or 650 mass intervals suggested that MPIase contains multiple units of these sizes. Thus, we picked up fragment ions at m/z 608 or 650 in the MS spectrum. MS/MS analyses of the peak at m/z 608 showed that it consists of three components of 187, 203 and 217 mass units ( Fig. 1b , bottom), suggesting that MPIase contains repeating trisaccharide units. From the results of composition analysis, the 203 mass unit component was attributed to N -acetyl-glucosamine (GlcNAc) in the dehydrated form. GlcNAc residues are non-stoichiometrically O -acetylated, because another building block of 245 mass unit was detected instead of 203 in MS/MS spectra of the peak at m/z 650 ( Supplementary Fig. S4 ). The other building blocks of 187 and 217 mass units were presumed to be N -acetyl-aminodeoxyhexose and N -acetyl-aminohexuronic acid, respectively. The calculated masses (averages of isotopic isomers) of the estimated trisaccharide units are 607.56 (hydroxyl form: C 24 H 37 N 3 O 15 ) and 649.60 (acetoxy form: C 26 H 39 N 3 O 16 ), whereas the observed values were 607.9±0.6 and 649.9±0.7, respectively. Extensive two-dimensional nuclear magnetic resonance (2D NMR) analysis of MPIase supported that MPIase is composed of trisaccharide repeating units and a lipid moiety ( Fig. 1c ). Three amide protons that were additionally observed on 1 H-NMR in H 2 O ( Supplementary Fig. S5 ) proved that three acetamidosugars are present in each unit. On the basis of the cross-peak between the methyl signal at δ 1.10 and one of the amide protons in a rotating-frame nuclear Overhauser effect correlation spectroscopy (ROESY) spectrum, 4-acetamido-4-deoxyfucose (Fuc4NAc) was assumed to be a candidate aminodeoxyhexose. On comparison of the peak intensity of the methyl group at δ 1.10 and that of the O -acetyl group at δ 2.21, about 1/3 of the GlcNAc residues were estimated to be O -acetylated. The glycan and lipid parts of MPIase were cleaved through mild hydrolysis with 48% aqueous hydrogen fluoride (HF) to give a hydrophilic fraction (HF-MPIase). Methanolysis of HF-MPIase gave three major peaks on GC–MS ( Fig. 2a ), one of which proved to be GlcNAc. Another one was identified with synthesized authentic Fuc4NAc ( Supplementary Fig. S6 and Supplementary Methods ). The remaining peak was unequivocally assigned as 2-acetamido-2-deoxymannuronic acid (ManNAcA) through comparison with some synthetic authentic uronic acids ( Supplementary Fig. S7 ). All sugars have the D-configuration, as proved on GC–MS analyses of the glycosides obtained on solvolysis in ( S )-(+)-2-butanol [13] . 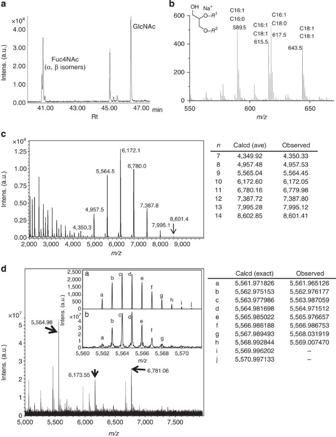Figure 2: Structure determination of hydrolysed MPIase derivatives. (a) GC–MS of methanolysis products of HF-MPIase after peracetylation. Three peaks were mainly observed in a total ion current (TIC) chromatogram, which were assigned as Fuc4NAc, ManNAcA and GlcNAc, respectively, on comparison with synthesized specimens. (b) Q-TOF MS of the hydrophobic fraction obtained on HF hydrolysis. DAGs possessing the designated fatty acids were detected as Na+adduct ions. (c, left) MALDI-TOF MS spectrum of NaOH-MPIase in the negative mode. (Right) The observedm/zvalues and calculated masses (averages of isotopic isomers) are compared. (d, left) MALDI-FT-ICR MS spectrum of NaOH-MPIase in the negative mode. The mass detection was focused on the high-mass range over 5 kDa. (Inset) The expanded spectrum aroundm/z5,565. (a) The calculated spectrum for the chemical formula C216H335N27O139P. (b) The accurate mass spectrum of the NaOH-MPIase atm/z5,565. (Right) Comparison of calculated masses and observed values. a.u., arbitrary unit. Figure 2: Structure determination of hydrolysed MPIase derivatives. ( a ) GC–MS of methanolysis products of HF-MPIase after peracetylation. Three peaks were mainly observed in a total ion current (TIC) chromatogram, which were assigned as Fuc4NAc, ManNAcA and GlcNAc, respectively, on comparison with synthesized specimens. ( b ) Q-TOF MS of the hydrophobic fraction obtained on HF hydrolysis. DAGs possessing the designated fatty acids were detected as Na + adduct ions. ( c , left) MALDI-TOF MS spectrum of NaOH-MPIase in the negative mode. (Right) The observed m/z values and calculated masses (averages of isotopic isomers) are compared. ( d , left) MALDI-FT-ICR MS spectrum of NaOH-MPIase in the negative mode. The mass detection was focused on the high-mass range over 5 kDa. (Inset) The expanded spectrum around m/z 5,565. (a) The calculated spectrum for the chemical formula C 216 H 335 N 27 O 139 P. (b) The accurate mass spectrum of the NaOH-MPIase at m/z 5,565. (Right) Comparison of calculated masses and observed values. a.u., arbitrary unit. Full size image Reduction of the terminal sugar of HF-MPIase gave 2-amino-2-deoxyglucitol, indicating that the reducing terminal is GlcNAc. The sequence and linkage mode of the trisaccharide were determined by 2D NMR of HF-MPIase. All signals on 1 H- and 13 C-NMR were assigned based on the 1 H double quantum filtered-correlation spectroscopy (DQF-COSY), total correlation spectroscopy (TOCSY), nuclear Overhauser enhancement spectroscopy (NOESY), ROESY, 1 H{ 13 C}HSQC (heteronuclear single quantum coherence) and 1 H{ 13 C}HMBC (heteronuclear multiple-bond correlation) results ( Supplementary Fig. S8–S13 and Supplementary Table S1 ). The correlation peaks observed on 1 H{ 13 C}HMBC suggested the glycosidic linkage of ManNAcA and Fuc4NAc ( Supplementary Fig. S13 ), but the linking position on GlcNAc and the anomeric configuration of ManNAcA could not be determined. Therefore, we synthesized several model disaccharides ( Supplementary Figs. S14 and S15 ) and compared their 13 C-NMR spectra with that of HF-MPIase ( Supplementary Table S1 ), which unequivocally led to the conclusion that the repeating trisaccharide is →3)-α- D -Fuc4NAc-(1→4)-β- D -ManNAcA-(1→4)-α- D -GlcNAc-(1→. Furthermore, a minor signal of the intact MPIase showed the presence of 6- O -acetylated GlcNAc. Quadrupole time-of-flight mass spectrometry (Q-TOF MS) of the hydrophobic fraction obtained on HF hydrolysis gave peaks of DAG ( Fig. 2b ). Fatty acids of 16:0, 16:1, 18:0 and 18:1, which are typical of E. coli lipids [14] , were observed, although fatty acid analyses by GC–MS indicated that their ratio varied with the culture lot. The presence of two phosphorus atoms was demonstrated on 31 P-NMR of MPIase ( Fig. 1d ), which were assigned as a pyrophosphate diester from their characteristic chemical shifts (−11.3 and −13.0 ppm) [15] . A cross-peak between one of the phosphorus signals and a small signal in the anomeric proton region in the 1 H{ 31 P}HMBC spectrum indicated that the reducing terminal of the glycan is linked to a pyrophosphate moiety ( Supplementary Fig. S16 ). The other phosphorus signal was correlated with the glycerol linker. Moreover, after hydrolysis of MPIase with cold NaOH followed by partitioning (NaOH-MPIase), only one 31 P peak was observed at 1.5 ppm, demonstrating the cleavage of the pyrophosphate to yield a monophosphate. The number of repeating trisaccharide units was determined by MALDI–TOF MS of NaOH-MPIase, because it gave a simpler MS spectrum owing to the loss of the lipid and O -acetyl moieties ( Fig. 2c ). The intense ions ( m/z 5,565, 6,172 and 6,780) correspond to n =9–11, whereas those of intact MPIase seemed to correspond to n =8–10 considering the lipid and O -acetyl moieties ( Fig. 1b ). The highest-mass peak in the spectrum of NaOH-MPIase was observed at m/z 8,601, corresponding to n =14, which was a higher molecular size than that of the highest-mass peak ( m/z ~7,600) observed in the spectrum of intact MPIase ( Fig. 1b ). These apparent discrepancies can be explained by the higher ionization efficiency of the phosphate ion moiety in NaOH-MPIase. The enhanced ionization improved the quality (S/N ratio) of spectra, the effect being more evident in higher mass ranges. The observed regular intervals with 608 mass units suggest that MPIase is a mixture of homologous molecules with different numbers of repeating units in the glycan part. There is at moment no definite evidence to exclude the possibility that MPIase has a longer chain ( n >14) and that the fragment ions from the same parent glycan are generated in the ionization process to give the observed series of peaks. We concluded, however, that these are not the case from the following consideration: fragmentations in the ionization process would occur at any glycosidic linkages leading to a more complex MS pattern. Peaks under m/z 4,000, which show irregular intervals, are attributed to fragment ions yielded during the ionization. It is most likely that the glycan with various length are biogenetically generated and the abundant species are n =9–11. Finally, we succeeded in the detection of isotopic isomers at one of the peaks ( m/z 5,565) of NaOH-MPIase with sufficiently high resolution by MALDI Fourier transform ion cyclotron resonance mass spectrometry (MALDI-FT-ICR MS) in the high-mass range (>5 kDa) ( Fig. 2d ). The accurate masses of the isotopic peaks indicate the chemical formula C 216 H 335 N 27 O 139 P, which corresponds to the nine trisaccharide repeating units with a monophosphate. When the mass detection was focused on the middle- to high-mass range around 3 kDa, fragment ions of a glycan without a phosphate moiety were detected ( Supplementary Fig. S17 ). The mass difference of 607.2 was well coincident with the chemical formula C 24 H 37 N 3 O 15 (calculated accurate mass, 607.223), corresponding to one repeating unit of NaOH-MPIase. Taking the aforementioned information into account, we determined the structure of MPIase to be as shown in Fig 1a . Surprisingly, the trisaccharide unit of MPIase is similar to the reported structure of enterobacterial common antigen (ECA), an outer membrane constituent [16] , [17] , [18] , [19] ( Supplementary Table S1 ), although ECA has a monophosphate linker instead of the pyrophosphate in MPIase ( Fig. 3a ). The number of repeating units in MPIase was mainly 9–11, whereas that in ECA was reported to be 18–55 (refs. 16 , 17 ). 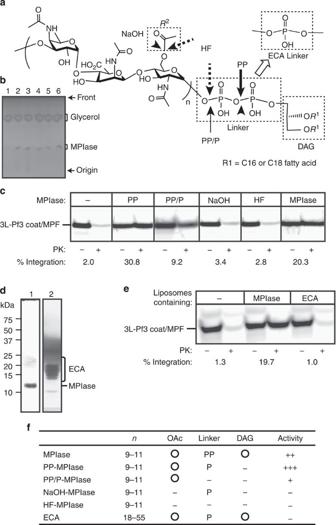Figure 3: Structure–activity relationship. (a) The positions of the digestions are indicated by a solid arrow (PP-MPIase), a light arrow (PP/P-MPIase), arrowheads (NaOH-MPIase) and dotted arrows (HF-MPIase). (b) The MPIase derivatives, dissolved at 1 mg ml−1in buffer A (50 mM HEPES-KOH (pH 7.5), 10% glycerol) were analysed by TLC/anisaldehyde-H2SO4staining. Two microliters each of buffer A (lane 1), PP-MPIase (lane 2), PP/P-MPIase (lane 3), NaOH-MPIase (lane 4) and HF-MPIase (lane 5) were spotted. In lane 6, MPIase (2 μg) and buffer A (2 μl) were also spotted. The positions of MPIase derivatives, glycerol and the front/origin are indicated at the right. (c) Integration activities of 3L-Pf3 coat in the presence of liposomes (0.4 mg ml−1) and the indicated MPIase derivatives (50 μg ml−1). Considering the average molecular weight of MPIase to be ~7,000, the concentrations of PP-MPIase, PP/P-MPIase, NaOH-MPIase and HF-MPIase were 7.9, 8.0, 8.0 and 8.1 μM, respectively. Undigested MPIase (MPIase, 7.1 μM), reconstituted as reported11, was also analysed. The integration activities are indicated as percentages as to synthesized 3L-Pf3 coat. (d) Purified preparations (3 μg) of MPIase (lane 1) and ECA (lane 2) were analysed by SDS–PAGE/silver staining. The positions of each material and molecular weight markers are indicated at the right and left, respectively. (e) Liposomes, into which MPIase and ECA had been reconstituted at 5% of phospholipids, were subjected to the 3L-Pf3 coat integration assay. The integration activities are indicated. (f) Summary of the structures and activities of MPIase derivatives and ECA. The numbers of glycan repeating units (n), and the presence of OAc groups, the linker (PP, pyrophosphate; P, phosphate) and DAG are shown. The integration activity of each material was evaluated from −to +++. Figure 3: Structure–activity relationship. ( a ) The positions of the digestions are indicated by a solid arrow (PP-MPIase), a light arrow (PP/P-MPIase), arrowheads (NaOH-MPIase) and dotted arrows (HF-MPIase). ( b ) The MPIase derivatives, dissolved at 1 mg ml −1 in buffer A (50 mM HEPES-KOH (pH 7.5), 10% glycerol) were analysed by TLC/anisaldehyde-H 2 SO 4 staining. Two microliters each of buffer A (lane 1), PP-MPIase (lane 2), PP/P-MPIase (lane 3), NaOH-MPIase (lane 4) and HF-MPIase (lane 5) were spotted. In lane 6, MPIase (2 μg) and buffer A (2 μl) were also spotted. The positions of MPIase derivatives, glycerol and the front/origin are indicated at the right. ( c ) Integration activities of 3L-Pf3 coat in the presence of liposomes (0.4 mg ml −1 ) and the indicated MPIase derivatives (50 μg ml −1 ). Considering the average molecular weight of MPIase to be ~7,000, the concentrations of PP-MPIase, PP/P-MPIase, NaOH-MPIase and HF-MPIase were 7.9, 8.0, 8.0 and 8.1 μM, respectively. Undigested MPIase (MPIase, 7.1 μM), reconstituted as reported [11] , was also analysed. The integration activities are indicated as percentages as to synthesized 3L-Pf3 coat. ( d ) Purified preparations (3 μg) of MPIase (lane 1) and ECA (lane 2) were analysed by SDS–PAGE/silver staining. The positions of each material and molecular weight markers are indicated at the right and left, respectively. ( e ) Liposomes, into which MPIase and ECA had been reconstituted at 5% of phospholipids, were subjected to the 3L-Pf3 coat integration assay. The integration activities are indicated. ( f ) Summary of the structures and activities of MPIase derivatives and ECA. The numbers of glycan repeating units ( n ), and the presence of OAc groups, the linker (PP, pyrophosphate; P, phosphate) and DAG are shown. The integration activity of each material was evaluated from −to +++. Full size image Relationship between the structure and function of MPIase To clarify the relationship between its structure and function, MPIase was derivatized chemically and enzymatically ( Fig. 3 ). Pyrophosphatase ( Fig. 3a , solid arrow) or alkaline phosphatase in addition (light arrow) cleaved the linkage without loss of the O -acetyl groups to give pyrophosphatase-treated MPIase (PP-MPIase) or pyrophosphatase/phosphatase-treated MPIase (PP/P-MPIase), respectively. By contrast, NaOH (arrowheads) or HF (dotted arrows) hydrolysed not only the linkage but also the O -acetyl groups to give NaOH-MPIase or HF-MPIase, respectively. These digestions generated soluble glycan chains devoid of the lipid moiety, which were analysed by thin-layer chromatography (TLC) to confirm their recovery ( Fig. 3b ). Then, their activities were determined by means of a model substrate, 3L-Pf3 coat protein [20] , [21] , [22] , of which integration is absolutely dependent on MPIase [10] , [11] ( Supplementary Fig. S18 ). PP-MPIase, added as a soluble factor to the integration reaction mixture, was more active as to 3L-Pf3 coat integration than authentic MPIase reconstituted into liposomes ( Fig. 3c ), indicating that the lipid part of MPIase is not essential for its function. A titration experiment confirmed these results even though it is assumed that theoretically half of the MPIase used for reconstitution was exposed on the outer surface of liposomes ( Supplementary Fig. S19 ). PP/P-MPIase retained weaker but definite activity ( Fig. 3c ). On the other hand, both NaOH-MPIase and HF-MPIase were inactive ( Fig. 3c ), indicating that the O -acetyl groups are essential for the function. The glycan chains of ECA are similar to but longer than those of MPIase [16] , [17] , [18] , [19] . We therefore examined whether or not ECA is involved in protein integration. ECA, prepared from outer membranes, gave a typical ladder, whereas purified MPIase gave a single band that is different from that of ECA on a silver-stained gel ( Fig. 3d ). When subjected to the integration assay, ECA was found to be completely inactive as to integration ( Fig. 3e ). These results suggest that the glycan chain length is important for integration. The structure–function relationship of MPIase is summarized in Fig 3f . MPIase possesses integration-dedicated chaperone-like activity Protein integration into membranes is a co-translational process even for Sec/SRP-independent proteins [1] , [2] . Hence, we examined whether or not this is the case in the presence of the soluble and active version of MPIase (PP-MPIase) ( Fig. 4a ). A co-translational mixture of both liposomes and PP-MPIase caused 3L-Pf3 coat integration (co/co), whereas post-translational addition of PP-MPIase did not (co/post). Integration into liposomes that had been post-translationally added could hardly be detected when PP-MPIase was missing (post/−) or added post-translationally (post/post). By contrast, when PP-MPIase was present during translation, 3L-Pf3 coat was obviously integrated into post-translationally added liposomes (post/co), this being indicative of post-translational integration. In the absence of liposomes, 3L-Pf3 coat was digested on proteinase treatment irrespective of the presence (−/co) or absence (−/−) of PP-MPIase. These results suggest that PP-MPIase maintains the integration-competent structure through direct binding to 3L-Pf3 coat. This idea was further verified by means of gel filtration ( Fig. 4b–d ). Under the conditions used, PP-MPIase (~6.3 kDa) was eluted at around 50 kDa ( Fig. 4b ), suggesting that MPIase forms an octamer. When the translation mixture without PP-MPIase was applied, 3L-Pf3 coat (~5 kDa; Supplementary Fig. S18b ) was eluted at the void volume due to aggregation ( Fig. 4c ; −PP-MPIase). When PP-MPIase was present during translation, the majority of 3L-Pf3 coat shifted to fractions of lower molecular weight (+PP-MPIase) with a peak at ~160 kDa ( Fig. 4d ), indicating that PP-MPIase forms a soluble complex with 3L-Pf3 coat that is integration-competent, similar to the chaperone–TA membrane protein complex in eukaryotes [6] , [7] , [8] . The addition of an E. coli cytosolic fraction to the integration reaction mixture neither affected the MPIase-dependent integration nor caused spontaneous integration into DAG-containing liposomes, whereas it caused a slight increase in spontaneous integration into DAG-lacking liposomes ( Supplementary Fig. S20a,b ). When 3L-Pf3 coat synthesized in the presence of cytosol was analysed by gel filtration, a significant amount of 3L-Pf3 coat was solubilized presumably by cytosolic chaperones ( Supplementary Fig. S20c,d ). These results suggest that there are no factors present in the cytosol that possess integration-dedicated chaperone activity or protein integrase activity. Taking these results together, we concluded that MPIase possesses integration-dedicated chaperone-like activity. 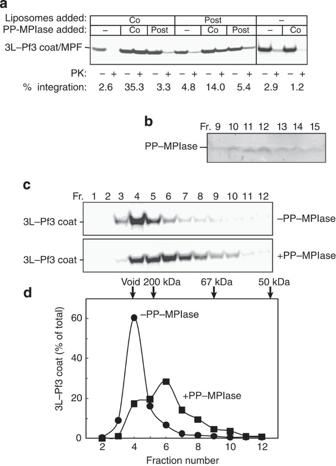Figure 4: Integration-dedicated chaperone-like activity of MPIase. (a) 3L-Pf3 coat was synthesized in the presence (co) or absence (post and −) of liposomes or PP-MPIase (50 μg ml−1). After 30 min incubation at 37 °C, translation was terminated by the addition of chloramphenicol (25 μg ml−1), and the reaction mixtures were incubated for 5 min at 37 °C. To some samples, PP-MPIase and/or liposomes were added, and then the reaction mixtures were further incubated for 30 min at 37 °C (post), whereas other samples were subjected to proteinase K digestion. The integration activity of each sample is indicated. (b) PP-MPIase (10 μg in 50 μl of buffer A) was applied to a Superose 12 column, which had been equilibrated with 50 mM HEPES-KOH (pH 7.5). The column was developed at 1.0 ml min−1and 0.5 ml fractions were collected from 5 min after the start. An aliquot (100 μl) of each fraction was precipitated with acetone (80%), followed by analysis by TLC/anisaldehyde-H2SO4staining. The position of PP-MPIase is indicated. (c) The translation mixture of 3L-Pf3 coat (50 μl) in the presence (bottom) and absence (top) of PP-MPIase (200 μg ml−1) was applied to a Superose 12 column. The column was developed and fractions were collected as inb. An aliquot of each fraction (100 μl) was precipitated with TCA (5%), followed by analysis by SDS–PAGE/autoradiography. The position of 3L-Pf3 coat is indicated. (d) The amount of 3L-Pf3 coat in each fraction incwas determined and is plotted as a percentage of the total amount. Figure 4: Integration-dedicated chaperone-like activity of MPIase. ( a ) 3L-Pf3 coat was synthesized in the presence (co) or absence (post and −) of liposomes or PP-MPIase (50 μg ml −1 ). After 30 min incubation at 37 °C, translation was terminated by the addition of chloramphenicol (25 μg ml −1 ), and the reaction mixtures were incubated for 5 min at 37 °C. To some samples, PP-MPIase and/or liposomes were added, and then the reaction mixtures were further incubated for 30 min at 37 °C (post), whereas other samples were subjected to proteinase K digestion. The integration activity of each sample is indicated. ( b ) PP-MPIase (10 μg in 50 μl of buffer A) was applied to a Superose 12 column, which had been equilibrated with 50 mM HEPES-KOH (pH 7.5). The column was developed at 1.0 ml min −1 and 0.5 ml fractions were collected from 5 min after the start. An aliquot (100 μl) of each fraction was precipitated with acetone (80%), followed by analysis by TLC/anisaldehyde-H 2 SO 4 staining. The position of PP-MPIase is indicated. ( c ) The translation mixture of 3L-Pf3 coat (50 μl) in the presence (bottom) and absence (top) of PP-MPIase (200 μg ml −1 ) was applied to a Superose 12 column. The column was developed and fractions were collected as in b . An aliquot of each fraction (100 μl) was precipitated with TCA (5%), followed by analysis by SDS–PAGE/autoradiography. The position of 3L-Pf3 coat is indicated. ( d ) The amount of 3L-Pf3 coat in each fraction in c was determined and is plotted as a percentage of the total amount. Full size image Subcellular localization of MPIase We then examined the subcellular localization of MPIase by means of anti-MPIase antibodies (αMPIase). Immunoblot analysis revealed that MPIase is localized in inner membranes ( Fig. 5a ), as expected. Successful cell fractionation was confirmed by the appearance of the respective marker proteins ( Fig. 5b–d ). The ECA ladder was detected when each fraction was prepared from the wild-type strain because of the similarity of the glycans ( Fig. 5a ). Unlike the precursor form of ECA found in inner membranes, the mature ECA in outer membranes was hardly detected [16] . Only MPIase, that is, not the ECA ladder, was detected for the inner membrane fraction prepared from the wecA ( rfe ) mutant [23] , an ECA-deficient strain ( Fig. 5a ). These results indicate that the biosynthetic pathway for MPIase is different from that for ECA. 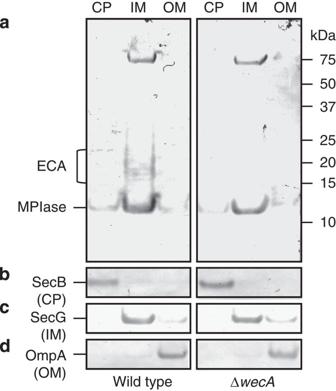Figure 5: Subcellular localization of MPIase. (a) MPIase was detected on immunoblots41of cytoplasm/periplasm (CP), inner membranes (IM) and outer membranes (OM) from MC4100 (ref.42) (wild type, left) and JW375843(ΔwecA, right). A band of ~72 kDa was also detected for IM. SecB, a cytosolic protein (b), SecG, an inner membrane protein (c) and OmpA, an outer membrane protein (d) were also detected to confirm the successful fractionation. Figure 5: Subcellular localization of MPIase. ( a ) MPIase was detected on immunoblots [41] of cytoplasm/periplasm (CP), inner membranes (IM) and outer membranes (OM) from MC4100 (ref. 42 ) (wild type, left) and JW3758 [43] (Δ wecA , right). A band of ~72 kDa was also detected for IM. SecB, a cytosolic protein ( b ), SecG, an inner membrane protein ( c ) and OmpA, an outer membrane protein ( d ) were also detected to confirm the successful fractionation. Full size image Anti-MPIase IgG inhibits protein integration into native INV Application of this antibody allowed us to prove the importance of MPIase for integration into native INV. αMPIase immunoglobulin G (IgG) clearly inhibited 3L-Pf3 coat integration into liposomes containing either MPIase or PP-MPIase ( Fig. 6a ), and in the presence of cytosol as well ( Supplementary Fig. S20a ). When αMPIase IgG was incubated with INV prepared from wild-type cells, the integration activity was obviously inhibited to ~1/3 in a concentration-dependent manner ( Fig. 6b ). Similar inhibition was seen with smaller amounts of αMPIase IgG when ECA-deficient ( wecF / rffT [23] ) INV were used ( Fig. 6b ), suggesting that the ECA precursor competes with MPIase as to interaction with the antibody. These results clearly indicate that MPIase is operative in native INV as in model liposome systems. The weaker inhibition observed in INV presumably reflects the steric hindrance of SecYEG that cooperates with MPIase in Sec-dependent reactions [9] . 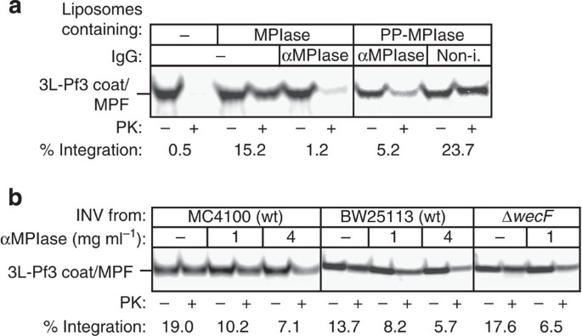Figure 6: Anti-MPIase IgG inhibits integration. (a) αMPIase or non-immune (non-i.) IgG was added to integration reaction mixtures at 1 mg ml−1together with MPIase-reconstituted liposomes or liposomes supplemented with PP-MPIase. (b) αMPIase IgG was added to integration reaction mixtures together with INV from MC4100 (wild type (wt)), BW25113 (wt) and JW5596 (ref.43) (BW25113 ΔwecF). The integration activity of 3L-Pf3 coat is indicated. Figure 6: Anti-MPIase IgG inhibits integration. ( a ) αMPIase or non-immune (non-i.) IgG was added to integration reaction mixtures at 1 mg ml −1 together with MPIase-reconstituted liposomes or liposomes supplemented with PP-MPIase. ( b ) αMPIase IgG was added to integration reaction mixtures together with INV from MC4100 (wild type (wt)), BW25113 (wt) and JW5596 (ref. 43 ) (BW25113 Δ wecF ). The integration activity of 3L-Pf3 coat is indicated. Full size image In this study, we have determined the complete structure of MPIase, analysed its function and studied its structure–function relationship. We demonstrated that MPIase, in spite of its non-proteinaceous architecture, is a new integration-dedicated chaperone-like molecule that drives subsequent protein integration into membranes. Although a number of functional molecules, including molecular chaperones, protein integrase and protein translocase, have been identified as factors participating in protein transport [1] , [2] , [3] , no glycolipid has been reported to have such a function. Stoichiometric analysis indicated that each MPIase caused the integration of higher numbers of 3L-Pf3 coat molecules [10] , that is, MPIase catalytically drives protein integration reactions, which never proceed in a spontaneous manner [9] , [10] , [21] . Moreover, the inhibition of protein integration by αMPIase antibodies indicates that MPIase is involved under physiological conditions. On the basis of these observations, we concluded that MPIase functions like an enzyme, leading us to propose the new concept of a ‘glycolipozyme’ for MPIase (see below). The function of MPIase can be dissected into two steps: the first is binding with a substrate protein for transport to membranes, and the second is its membrane integration. In the former step, MPIase captures membrane proteins and thereby prevents their aggregation, as revealed by the experiments involving PP-MPIase. It has been reported that GET factors (yeast) or Bat3 complex (mammal) act as chaperones in TA membrane protein targeting to endoplasmic reticulum membranes [5] , [6] , [7] , [8] , their functions being analogous to those of MPIase. In the case of the integration step, it may be possible that the chaperone-like activity of MPIase solubilized membrane proteins, providing more chances for spontaneous integration. However, this possibility seems unlikely because the DAG effect is potent enough to prevent spontaneous integration. In fact, partially solubilized 3L-Pf3 coat in the presence of E. coli cytosol did not cause integration into DAG-containing liposomes ( Supplementary Fig. S20 ). Moreover, we have reported that solubilized MtlA (mannitol permease), which is a Sec/SRP-dependent substrate chaperoned by SRP, was completely prevented from being integrated into DAG-containing liposomes, although it became significantly embedded into the DAG-lacking liposomes in a spontaneous manner [9] . Therefore, we concluded that the integration of 3L-Pf3 coat caused by MPIase was not due to the enhancement of spontaneous integration but to that MPIase actively integrates membrane proteins after capturing them. The function of MPIase apparently coincides with that of membrane protein integrase we have assumed. Thus, we conceived of the concept of a ‘glycolipozyme’ due to the enzyme-like activity of MPIase. In addition to the above-mentioned transport factors, YidC has been identified in E. coli as an important protein for integration [24] . YidC, homologous to mitochondrial Oxa1p and Albino 3 in chloroplasts [25] , can be efficiently crosslinked with nascent membrane proteins [26] , [27] in a manner similar to in the case of translocating chain-associating membrane (TRAM) protein [28] in the endoplasmic reticulum ( Supplementary Fig. S1 ). It is evident that YidC is involved in the biogenesis of membrane proteins ( Supplementary Fig. S2 ); however, there has been controversy as to whether or not YidC functions as a ‘membrane protein insertase’. Reconstitution of MtlA integration required SecYEG and MPIase but not YidC [9] . LacY (lactose permease) folding but not its membrane integration was severely affected by YidC depletion [29] , suggesting a membrane chaperone activity of YidC. Although reconstitution of integration of Sec/SRP-independent substrates has been reported to be YidC-dependent, spontaneous integration was not completely excluded in the reports [20] , [21] . On the other hand, the MPIase dependency as a membrane protein integrase was clearly demonstrated irrespective of whether the substrates were Sec/SRP-dependent or -independent ones, when artificial spontaneous integration was blocked by physiological concentrations of DAG [9] , [10] , [11] . Considering that YidC can be efficiently crosslinked with nascent membrane proteins [26] , [27] , it is likely that YidC functions at a late step of integration. MPIase would function in advance of YidC, and is thus more plausibly a membrane protein integrase. A working model for the MPIase- or PP-MPIase-dependent integration of 3L-Pf3 coat is illustrated in Fig. 7 . MPIase captures 3L-Pf3 coat on the membrane surface, keeping it soluble ( Fig. 7a , step 1). MPIase may form an oligomer on membranes, judged from the results of gel filtration of PP-MPIase ( Fig. 4b ). For the next integration step, we speculate that the structural change of MPIase associated with 3L-Pf3 coat (step 2) induces the transport of 3L-Pf3 coat into the bilayer, probably due to more hydrophobic interactions of membrane lipids (step 3), followed by completion of integration (step 4). At this step, YidC might assist integration. The released MPIase can function in the next cycle (step 5), explaining the catalytic role of MPIase. In the case of PP-MPIase ( Fig. 7b ), interaction between PP-MPIase and 3L-Pf3 coat occurs in the cytosol (step 0). After membrane targeting (step 1′), a similar structural change to MPIase (step 2′) allows integration (steps 3′ and 4′). The released PP-MPIase functions in the next step (step 5′) like MPIase. The capture of 3L-Pf3 coat in the soluble milieu explains the higher activity of PP-MPIase. 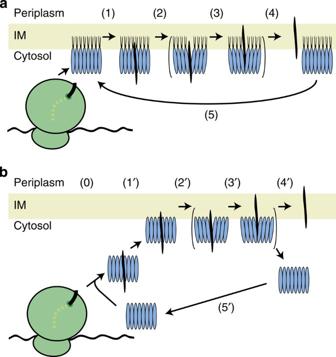Figure 7: Working model of 3L-Pf3 coat integration. Plausible mechanisms of MPIase- (a) and PP-MPIase- (b) dependent integration of 3L-Pf3 coat are shown. The oligomeric state of MPIase and steps in parentheses are speculative. For details, see text. Figure 7: Working model of 3L-Pf3 coat integration. Plausible mechanisms of MPIase- ( a ) and PP-MPIase- ( b ) dependent integration of 3L-Pf3 coat are shown. The oligomeric state of MPIase and steps in parentheses are speculative. For details, see text. Full size image Structure–function relationship studies revealed that the glycan chains are essential and sufficient for the integration. Of note is that the glycan of MPIase contains total 30–40 acetyl groups, which render the molecule hydrophobic overall and may facilitate its direct binding with membrane proteins. The importance of the acetyl groups is supported by the fact that MPIase is inactivated on the loss of the O -acetyl groups. The proteinase K-sensitivity of MPIase, which we previously showed [9] , could be explained by digestion of the amide bonds in N -acetyl groups, as the substrate specificity of proteinase K is very low [30] . The essential nature of the soluble glycan of MPIase devoid of the lipid moiety excludes the possibility that MPIase neutralizes the DAG effect to regain the spontaneous integration activity. It also indicates that MPIase functions at the cytoplasmic face of inner membranes. Outer membrane-associated ECA possessing similar but longer glycan chains was inactive in our study. It might be difficult for the longer chains to gain access to membranes. It has been reported that cyclic ECA, which contains four trisaccharide repeats of a cyclic form [31] , was found as an inseparatable contaminant of various proteins expressed in bacteria [32] . The glycan of MPIase is expected to interact with various membrane proteins, it exhibiting chaperone-like activity. Although the function of ECA remains totally unknown so far, the localization and biosynthetic precursors of MPIase and ECA are different. They must have evolved in different manners. In summary, we revealed that a new glycolipid MPIase functions like an enzyme as a membrane protein integrase. So far, the functions of glycans have been well studied, glycan–glycan and glycan–protein interactions being important for many cellular processes, such as cell identification, infection by pathogenic bacteria and viruses, signal transduction and so on [33] , [34] , [35] , [36] , [37] . However, the function of MPIase is rather different from such interactions. From this aspect, the structure–function analysis of MPIase not only allowed detailed characterization of the molecular mechanisms underlying membrane protein integration but also shed new light on glycolipid biology. Materials MPIase was purified from MC4100 as described [11] . INV [9] and reconstituted liposomes containing DAG [11] were prepared as described. The anti-MPIase antibodies were raised in a rabbit against purified MPIase [11] crosslinked to keyhole limpet hemocyanin. ECA was prepared from MC4100 as described [38] . Amino-acid analysis MPIase (100 μg) was hydrolysed with 6 M HCl (100 μl at 100 °C for 20 h), and an aliquot (50 μl) was labelled with AccQ-TagTM (Waters) for HPLC analysis. NMR study NMR spectra were measured at 298 K on either a Bruker AVANCE-750 equipped with a cryoprobe ( 1 H resonance frequency: 750.13 MHz) or a Bruker DMX-500 ( 1 H resonance frequency: 500.13 MHz). A sample (1.0 mg) was dissolved in 170 μl of D 2 O or 5% D 2 O/H 2 O and then placed in a Shigemi tube made of a special type of glass with magnetic susceptibility matching to that of the solvent. Chemical shifts are reported in ppm relative to the solvent peak (H 2 O: δ=4.80) for 1 H-NMR, external 3-trimethylsilyl-1-propionic acid in D 2 O (δ=0.0) for 13 C-NMR or external 5% aqueous H 3 PO 4 (δ=0.0) for 31 P-NMR. Two-dimensional spectroscopic data were processed by XWINNMR software (Bruker Biospin). MALDI–TOF MS analyses MS spectra were measured on Bruker Ultraflex III MALDI–TOF/TOF MS. A sample (300 μg) was dissolved in 100 μl of 20% EtOH. 2,5-Dihydroxy benzoic acid dissolved in 20% EtOH at 10 mg ml −1 final concentration was used as a matrix. The sample and matrix were mixed in a 1:2 ratio, and then the mixed solution was deposited on the target plate. Peaks were detected in the negative-liner mode and calibrated with external peptide standards. The MS/MS spectrum was analysed in the positive-reflecting mode and calibrated with CsI as an external standard. MALDI–FT–ICR MS analyses Ultra-high-resolution mass spectra were acquired with a Solarix 7.0T FT–ICR–MS equipped with a electrospray ionization/MALDI dual ion source (Bruker Daltonics). The exact mass spectra were calibrated with the signal of insulin as the internal standard after the spectra had been calibrated with the nucleotide calibration standards as the external standards. A sample (200 μg) was dissolved in a 60 μl aqueous solution (CHCl 3 :MeOH:H 2 O=3:7:4), and 2,5-dihydroxy benzoic acid in 20% EtOH was used as a matrix. Hydrolysis of MPIase MPIase was hydrolysed with 1 M NaOH in 20% MeOH (4 °C for 22 h) or 48% aqueous HF (4 °C for 48 h), followed by partitioning with CHCl 3 /MeOH/H 2 O (3/2/1). The aqueous phase was lyophilized to give NaOH-MPIase and HF-MPIase, respectively. Constitutive sugar analysis HF-MPIase or an authentic sugar (100 μg) was subjected to methanolysis (5% HCl/MeOH, 85 °C for 23 h, under an Ar atmosphere) before peracetylation (acetic anhydride/pyridine: 50 μl/50 μl at 100 °C for 30 min, under an Ar atmosphere). The mixture was concentrated in vacuo and the residue was dissolved in CHCl 3 (500 μl), which was washed twice with water (500 μl), followed by a concentration in vacuo . The residue was dissolved in CH 2 Cl 2 (100 μl) and then an aliquot (1 μl) was analysed on a GC–MS system in the split injection mode, with a split ratio of 1:10. GC–MS analysis was performed on an Network GC system 6890 N connected to an Inert Mass Selective Detector 5975 (Agilent Technologies) using He as the carrier gas and an HP-5 ms capillary column (30 m × 0.25 mm i.d., 0.25 μm d.f.) operating with the following temperature programme: 40 °C (10 min)−5 °C min −1 −250 °C (30 min). Fatty acid analysis The methanolysis products of MPIase (100 μg) with 5% HCl/MeOH (1.0 ml at 100 °C for 2 h, under an Ar atmosphere) were dissolved in CH 2 Cl 2 (100 μl), and an aliquot (1 μl) was subjected to GC–MS. MPIase (300 μg) was hydrolysed with 48% aqueous HF, followed by partition with CHCl 3 /MeOH/H 2 O (3/2/1). The organic phase was concentrated and the residue was dissolved in MeOH (40 μl). An aliquot (5 μl) was further diluted in MeOH (45 μl), followed by Q–TOF–MS (Micromass). Electrospray ionization MS was performed in the positive mode with aqueous MeOH as the mobile phase. Digestion of MPIase The pyrophosphatase (Sigma; 0.5 mg ml −1 ) and alkaline phosphatase (Takara; 20 U ml −1 ) digestions were performed for 3 h at 37 °C and 65 °C, respectively, followed by recovery of the products by acetone (80%) precipitation. MPIase and its derivatives were analysed by SDS–polyacrylamide gel electrophoresis (PAGE)/silver staining or TLC/anisaldehyde-H 2 SO 4 staining [11] . Integration assay Integration of 3L-Pf3 coat [22] ( Supplementary Fig. S18a,b ) was determined by protease protection assaying as described [11] ( Supplementary Fig. S18c ). After the translation reaction (20 μl) involving the pure system [11] , [39] , [40] in the presence of liposomes or INV (0.4 mg ml −1 ) had been carried out for 30 min at 37 °C, an aliquot (15 μl) was digested with proteinase K (0.5 mg ml −1 ), followed by trichloroacetic acid (TCA) precipitation, whereas an undigested sample (3 μl) was directly treated with TCA. Both samples were subjected to SDS–PAGE/autoradiography, followed by quantification of the membrane-protected fragments using a phosphorimager. How to cite this article: Ken-ichi N, et al . MPIase is a glycolipozyme essential for membrane protein integration. Nat. Commun. 3:1260 doi: 10.1038/ncomms2267 (2012).